Genome-wide RNAi ionomics screen reveals new genes and regulation of human trace element metabolism Trace elements are essential for human metabolism and dysregulation of their homoeostasis is associated with numerous disorders. Here we characterize mechanisms that regulate trace elements in human cells by designing and performing a genome-wide high-throughput siRNA/ionomics screen, and examining top hits in cellular and biochemical assays. The screen reveals high stability of the ionomes, especially the zinc ionome, and yields known regulators and novel candidates. We further uncover fundamental differences in the regulation of different trace elements. Specifically, selenium levels are controlled through the selenocysteine machinery and expression of abundant selenoproteins; copper balance is affected by lipid metabolism and requires machinery involved in protein trafficking and post-translational modifications; and the iron levels are influenced by iron import and expression of the iron/haeme-containing enzymes. Our approach can be applied to a variety of disease models and/or nutritional conditions, and the generated data set opens new directions for studies of human trace element metabolism. Trace elements are involved in most biological processes and are used by all living organisms. They serve as essential components of numerous proteins that carry out oxidation and reduction reactions, facilitate receptor activation and signalling events, participate in electron transfer, maintain structural integrity of proteins and have numerous other functions [1] , [2] , [3] . It is believed that one-third of human proteins bind metal ions [4] . Changes in trace element utilization and homoeostasis have been linked to many disorders. For example, mutations in the ATP7A gene are associated with low copper levels in most tissues and lethal disorder known as Menkes disease [5] . Mutations in the Wilson’s disease protein (ATP7B) result in a severe hepato-neurologic disorder due to accumulation of copper in the liver and brain [6] . Misbalance of other trace elements also causes serious disorders. For example, mutations in hepcidin and transferrin receptor 2 lead to iron overload and hereditary hemochromatosis [7] , whereas genetic defects in zinc transporter SLC39A4 are associated with acrodermatitis enteropathica, a disease of zinc deficiency. Available data indicate that the levels of trace elements, similar to levels of many metabolites, are kept within the narrow optimal range that is specific for each element and each tissue and cell type. Cells control trace elements through uptake, export, storage and compartmentalization, but relative roles of these processes vary for different trace elements, cell types, tissues and organisms. Several key components of the element-specific machineries have been identified, along with distinct modes of regulation, such as transcriptional control, regulation of protein stability, kinase-mediated phosphorylation and intracellular trafficking. For example, import of copper and iron in human cells is mediated predominantly by Ctr1 (Lee et al. [8] ) and the transferrin receptor system, respectively. The P-type ATPases ATP7A and ATP7B facilitate copper export, whereas ferroportin mediates iron efflux. Copper availability in the cytosol is controlled by metallochaperones (ATOX1, CCS and COX17) [1] , metallothioneins and the expression of copper-utilizing enzymes [9] . In contrast, cellular levels of iron are regulated at the level of messenger RNA for the iron storage molecule ferritin and for a key mediator of iron uptake transferrin receptor 1 (Barry et al. [10] and Theil [11] ). On the other hand, little is known about the uptake and export of selenium. This element is unique in that it is inserted into proteins co-translationally in the form of the 21st amino acid, selenocysteine (Sec), encoded by UGA codon. Such complex and energy demanding process most probably requires a tight regulation of intracellular selenium levels and recycling. The molecular machineries that regulate abundance and activity of key metal-handling molecules and fine-tune cellular ionomes remain mostly unknown [12] . Many regulators that control mRNA/protein stability, post-translational modification or intracellular trafficking are members of very large families of structurally related proteins (kinases, phosphatases and adaptor proteins), which make their identification challenging. Characterization of regulators at the level of individual proteins is time consuming and is mostly limited to molecules that are already known. In this regard, development of unbiased high-throughput assays could potentially address this problem. Recent years witnessed a remarkable expansion in high-throughput analyses, which take advantage of vast genomic resources. With regard to trace elements, these approaches somewhat lagged behind, in part due to challenges in analysing elements in small volumes and a high-throughput manner. Initial studies have been done with yeast [13] , [14] , [15] and plants [16] , paving a way to a new field, ionomics [17] , [18] , which aims to characterize trace element homoeostasis at the genome-wide level [16] , [19] , [20] , [21] . Here we use inductively coupled plasma mass spectrometry (ICP-MS) as the most sensitive method to analyse trace elements and develop an approach involving rapid element profiling coupled with the use of a human genome small interfering RNA (siRNA) library transfected into HeLa cells. Using this approach and the resulting ionomic data set, we aim to uncover previously uncharacterized regulators of trace element metabolism, which may serve as genetic markers for various nutritional conditions and disease states. A screen for genes that regulate human ionomes We developed and optimized a high-throughput method to analyse trace elements in mammalian cells (Methods). Among several cell lines subjected to initial tests, we had chosen HeLa cells for their high levels of most trace elements and reproducibility of ionome analyses. To control for changes in elemental composition, each plate included ATP7A siRNA as a positive control. Knockdown of ATP7A reproducibly increased cellular copper, as measured by ICP-MS in cell extracts ( Fig. 1a ) and by in situ X-ray fluorescence microscopy of fixed cells ( Fig. 1b ). The workflow ( Fig. 1c ) included the siRNA transfection, sample analysis, data processing, selection of the candidates for further analyses and validation studies. We employed a human siGenome SMARTPool siRNA library that targets 21,360 genes; this library was previously used in several genome-wide studies [22] . HeLa cells (~25,000 cells per well in a 96-well plate format) were transfected with pulled siRNA aliquots, each targeting a single gene (Methods). A fully robotic system was used for cell plating, growth, transfection and other manipulations, ensuring a high degree of consistency and precision. Following incubation and washing, cells were digested with the nitric acid/hydrogen peroxide mixture and analysed for levels of 18 elements by ICP-MS, which we custom equipped with a high-throughput sample delivery system. The levels of nine elements (selenium, copper, phosphorus, magnesium, potassium, cadmium, manganese, iron and zinc) were consistently above controls (samples without cells subjected to the same procedure); these nine elements were used, along with sodium and calcium, for further analysis. The method was optimized so that each sample was analysed in just over a minute. During a 3-month continuous run, each gene knockdown was analysed independently three times (that is, in three plates), and each sample (from each well) was assayed three times. This screen included more than two million measurements. 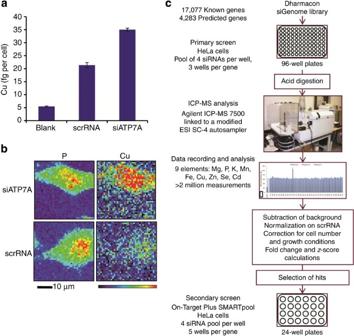Figure 1: Human genome-wide siRNA ionomics screen. (a) Effect of siRNA on copper levels in HeLa cells. Cells were transfected with human siATP7A, and 72 h after transfection, copper levels were analysed by ICP-MS. Error bars are onefold standard variances calculated from three replicates. (b) Impact of ATP7A deficiency on copper levels in HeLa cells. Cells were subjected to ATP7A knockdown as inaand examined by X-ray fluorescence microscopy. Scrambled RNA was used as control. Signals of copper and phosphorus are shown. The same single cell is shown in left and right panels. (c) siRNA ionomics screen. HeLa cells were transfected with the Human Genome SMARTpool Dharmacon siRNA library in 96-well plates followed by analysis of trace elements by ICP-MS. Concentrations of elements were analysed to obtain normalizedz-scores for each gene from the library and select primary hits. Figure 1: Human genome-wide siRNA ionomics screen. ( a ) Effect of siRNA on copper levels in HeLa cells. Cells were transfected with human siATP7A, and 72 h after transfection, copper levels were analysed by ICP-MS. Error bars are onefold standard variances calculated from three replicates. ( b ) Impact of ATP7A deficiency on copper levels in HeLa cells. Cells were subjected to ATP7A knockdown as in a and examined by X-ray fluorescence microscopy. Scrambled RNA was used as control. Signals of copper and phosphorus are shown. The same single cell is shown in left and right panels. ( c ) siRNA ionomics screen. HeLa cells were transfected with the Human Genome SMARTpool Dharmacon siRNA library in 96-well plates followed by analysis of trace elements by ICP-MS. Concentrations of elements were analysed to obtain normalized z -scores for each gene from the library and select primary hits. Full size image For data normalization, we used several approaches (Methods). The noise was first subtracted from the original signal for each knockdown sample. To account for changes in morphology, growth rate and size of cells caused by the siRNA treatment, we normalized the raw data to the average of four elements (phosphorus, manganese, selenium and zinc). The signals of these elements were most stable across the screen and therefore their average could be more accurately related to the amount of cells (than to the levels of any one element), especially if one of the normalization standards was affected. Second, to account for possible changes in instrument sensitivity over time as well as plate-to-plate variation, the data were normalized to the results obtained using the scrambled siRNA control on each plate. Finally, we generated the mean signal values of each gene from three replicates and calculated standard scores (also called z -scores, representing the number of s.d. from the mean; all z -scores are derived from three replicates) for each gene and each element to account for plate-to-plate variability. The positive control, ATP7A, z -scored at 9.49 and had the fifth highest score among the knockdown genes leading to copper elevation. APBA3 (an adaptor protein binding to β-amyloid A4 precursor protein) had the highest z -score of 14.25, although the effect of downregulation was not limited to copper. This result was nevertheless intriguing because previous reports indicated that β-amyloid A4 precursor protein was a copper-binding protein [23] . Most knockdowns that affected the levels of trace elements showed element-specific changes; ~3–5% of all analysed genes were affected ( z -score >5, Supplementary Fig. 1 ), with more hits (60–90%) corresponding to increases in element levels. To select significant knockdowns ( Supplementary Fig. 2 ), we checked the distributions of z -scores for each element and found that they were characterized by either normal or approximately normal distributions. To define the z -score threshold for each element, we calculated the prediction intervals for each element corresponding to the P value <0.05 (two tailed). We used the lower limit μ−1.96 δ , and upper limit μ+1.96 δ , where μ and δ represent the mean and the standard variation of z -scores for each element. The prediction intervals for each element were then used to build candidate lists by evaluating z -scores, which were beyond the prediction interval for each element. A total of 6,196 gene knockdowns (29%) were found to affect the levels of at least one element, with the majority of the knockdowns (4,051 genes) showing element-specific changes. We validated the selected gene candidates by retesting them in a 24-well format ( Table 1 ) to amplify the target element signal and validate the corresponding z -scores. We defined the z -score >3 as threshold and the z -score >5 as a guide for experimental analyses. Several of these genes encoded known regulators of trace element homoeostasis. For example, ATP7A and TFRC are the major players in the metabolism of copper and iron, respectively, and their downregulation altered levels of corresponding metals with z -scores of 9.49 and 7.1, respectively. All data have been summarized in the ionome database along with the tools that support data visualization and analysis for specific genes, accession numbers and screen plates ( http://www.gladyshevlab.bwh.harvard.edu/ICPMS_Human ). Table 1 Validated genes found to regulate trace elements in HeLa cells. Full size table Mechanisms of ionome regulation are element specific Analysis of the genes that affected elemental content of HeLa cells pointed to fundamental differences in the regulation of individual trace elements. For selenium, candidates with the highest z -scores included the selenoprotein thioredoxin reductase 1 (TR1) and a protein involved in Sec incorporation, SECIS-binding protein 2 (SBP2; Fig. 2a ). Interestingly, TR1 was the only selenoprotein whose knockdown dramatically decreased selenium levels, and SBP2 was the only member of the Sec insertion machinery that showed such effect ( Fig. 2b ). This finding suggests that SBP2 is a limiting factor in selenoprotein biosynthesis in HeLa cells and that selenoproteins represent a major pool of selenium in these cells. To clarify how the expression of just one selenoprotein (TR1) could alter selenium levels in HeLa cells, we metabolically labelled control and TR1-knockdown cells with 75 Se. This experiment revealed that TR1 was the most abundant selenoprotein in these cells, and that TR1 downregulation did not significantly affect the expression of other selenoproteins ( Fig. 2c ). Thus, the decreased expression of the most abundant selenoprotein was sufficient to alter selenium levels. Furthermore, we observed an excellent agreement between the abundance of individual selenoproteins and the effects of their knockdowns on total selenium levels. Altogether, the data suggested that the levels of selenium were affected by a key member of the Sec machinery and the expression of the most abundant selenoprotein. 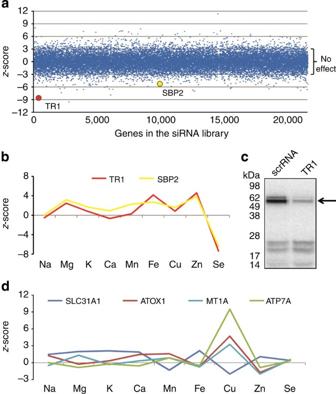Figure 2: Standard score analysis of targets identified in the ionomics screen in HeLa cells. (a) Distribution of selenium hits in the entire genome-wide human ionomics screen. Dots represent normalizedz-scores for each gene in the screen. Knockdowns of each gene in HeLa cells were analysed in triplicate. Knockdown phenotypes of TR1 and SBP2 are shown with coloured circles. (b) Ionomic profiles of TR1 and SBP2 obtained in the siRNA screen in HeLa cells. Note that only selenium signal changed significantly. (c)75Se metabolic labelling of HeLa cells with TR1 siRNA knockdown. HeLa cells were transfected with TR1 siRNA and scrRNA control, and metabolically labelled with75Se. Cell lysates were analysed by SDS–polyacrylamide gel electrophoresis, and the pattern of75Se labelling was visualized with a PhosphorImager. Migration of the TR1 band is shown with an arrow. (d) Ionomic profiles of siRNA gene knockdowns involved in copper metabolism.z-scores were obtained in the ionomic screen in HeLa cells. Figure 2: Standard score analysis of targets identified in the ionomics screen in HeLa cells. ( a ) Distribution of selenium hits in the entire genome-wide human ionomics screen. Dots represent normalized z -scores for each gene in the screen. Knockdowns of each gene in HeLa cells were analysed in triplicate. Knockdown phenotypes of TR1 and SBP2 are shown with coloured circles. ( b ) Ionomic profiles of TR1 and SBP2 obtained in the siRNA screen in HeLa cells. Note that only selenium signal changed significantly. ( c ) 75 Se metabolic labelling of HeLa cells with TR1 siRNA knockdown. HeLa cells were transfected with TR1 siRNA and scrRNA control, and metabolically labelled with 75 Se. Cell lysates were analysed by SDS–polyacrylamide gel electrophoresis, and the pattern of 75 Se labelling was visualized with a PhosphorImager. Migration of the TR1 band is shown with an arrow. ( d ) Ionomic profiles of siRNA gene knockdowns involved in copper metabolism. z -scores were obtained in the ionomic screen in HeLa cells. Full size image In general, the ionomes were stable, most notably the zinc ionome. On the other hand, for the iron ionome we detected many genes that mildly influenced the levels of several elements ( z -scores 3–4, based on three replicates). To evaluate which identified genes (and corresponding changes) might be physiologically relevant, we first considered consequences of downregulation of genes with a firmly established role in iron homoeostasis. Knockdown of TFRC decreased iron content ( z -score of 7.1), consistent with its key role in iron uptake, whereas downregulation of another known iron transporter, DMT2, was associated with a milder loss of cellular iron content ( z -score of 3.1). Although the transcripts with the z -scores between 2 and 3 did not pass the criteria of statistical threshold, several transcripts for proteins associated with iron metabolism were detected in this range of scores. For example, knockdown of iron-responsive element-binding protein 2 and δ-aminolevulinate synthase 2 (the first enzyme in the haeme synthesis pathway) yielded an increase in iron levels with the z -scores of 2.06 and 2.53, respectively, consistent with the previously reported biological effects of downregulation of these proteins [24] , [25] . Among iron-regulating genes with relatively high z -scores we detected ceruloplasmin, a ferroxidase, and huntingtin, a protein required for bioavailability of endocytosed iron [26] . Loss of either of these proteins in HeLa cells increased cellular iron levels ( z -scores of 3.2 and 3.9, respectively). In fact, downregulation of many iron- and haeme-containing enzymes was associated with iron elevation rather than deficiency. This observation suggests an exquisite sensing of total iron content and compensatory response, probably via an increased iron uptake. Given the observed range of z -scores for known regulators of iron homoeostasis (2.06–7.1), to identify cellular processes involved in iron balance we selected all genes, for which downregulation produced changes in the iron levels with a z -score above 3. Gene ontology analysis of this data set demonstrated that the most prominent biological process that influences Fe levels is the generation of precursor metabolites and energy ( Supplementary Table 1 ). The ontology analysis also revealed an important role of mitochondria in influencing iron metabolism, which is consistent with the role of this compartment in iron utilization for enzymatic reaction and formation of Fe-S clusters. In contrast to iron, copper levels showed much larger fluctuations. Although the number of genes affecting ionomes with lower z -scores (3–4) was similar for the iron and copper data sets, much larger number of genes altered copper content with z -scores above 4 compared with those for iron ( Supplementary Table 2 ). Several known regulators of copper metabolism caused copper elevation on knockdown with z -scores above 4: copper chaperone ATOX1 ( z -score of 4.7), metallothionein MT1A ( z -score of 4.27) and a copper-transporting ATPase ATP7A ( z -score of 9.4; Fig. 2d ). The difference between the iron and copper ionomes in the extent of fluctuations may be explained by the functionally different classes of molecules contributing to the balance of these elements. 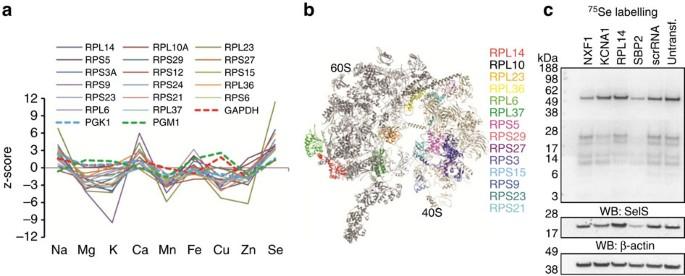Figure 3: Characterization of genes that affect the selenium ionome. (a) Ionomic profile data of the ribosomal functional cluster. Seleniumz-scores (derived from three replicates) from the screen were analysed by using DAVID. Glycolytic enzymes (GAPDH, PGK1 and PGM1) are shown for comparison. (b) Model of eukaryotic (yeast) 80S ribosome with the location of identified ribosomal cluster genes. (c) Analysis of selenium candidates in HeLa cells by metabolic75Se labelling. HeLa cells were transfected with the indicated siRNAs.75Se was added to the cells 24 h before harvesting. Cell lysates were analysed by SDS–polyacrylamide gel electrophoresis followed by western blotting with antibodies specific for selenoprotein S and β-actin. The75Se-labelling pattern was visualized with a PhosphorImager. Ontology analysis of the genes affecting copper levels with the z -scores higher than 4 pointed to endocytosis, RNA splicing and GTP hydrolysis as processes most frequently associated with altered copper metabolism and mostly distinct from those influencing Fe ionome ( Supplementary Table 3 ). 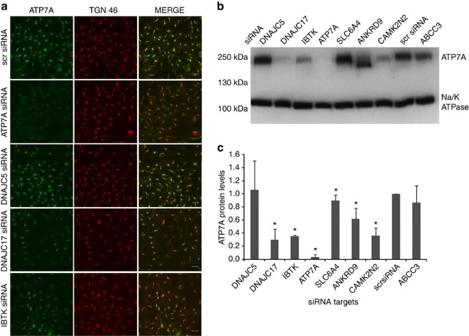Figure 4: Characterization of targets that affect copper levels in HeLa cells. (a) Effect of targets downregulation on ATP7A localization in basal conditions. Following gene-specific siRNA-mediated knockdowns, HeLa cells were fixed, stained with the antibodies against ATP7A (green) and the TGN marker TGN46 (red) and analysed by confocal microscopy. The merged image is shown in the right panel. Scale bar, 25 μm. (b) Effect of target downregulation on ATP7A protein levels and electrophoretic mobility. Following gene knockdowns, HeLa cell lysates were analysed by western blotting. The blot was cut at 130 kDa; the upper part was immunostained for ATP7A and the lower part was immunostained for Na/K-ATPase. A representative blot is shown; the entire blot is included asSupplementary Fig. 6. (c) Quantification of western blot data by densitometry. The ATP7A protein levels were normalized to Na/K-ATPase protein levels and the values were compared with the intensity of ATP7A in cells transfected with a non-targeting siRNA (scrRNA). The error bars correspond to s.d. values from four independent experiments. Asterisks mark significant changes (the Mann–WhitneyU-test,P<0.05; lower panel). Fifty-three genes were associated with the term ‘transport’; among those more than a half encoded proteins known to be involved in membrane protein trafficking ( Supplementary Table 4 ). We identified the γ-subunit of the adaptor-related protein complex 1 as a protein whose downregulation increased cellular copper content with a z -score of 5.09. This finding was especially exciting because, when this paper was in preparation, a mutation in another component of adaptor-related protein complex 1 was linked to a new disorder of copper metabolism [27] . Overall, our data suggested a fundamental role of trafficking processes in preventing copper overload. The data also enabled us to predict previously unidentified components of the secretory pathway associated with the copper export pathway. 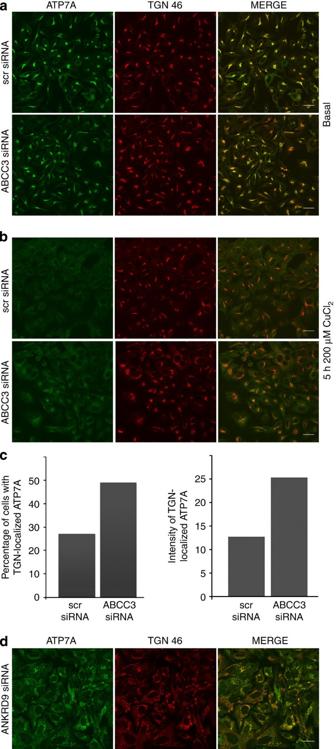Figure 5: ABCC3 and ANKRD9 are new regulators of ATP7A. (a–c) Downregulation of ABCC3 affects ATP7A trafficking. Following siRNA-mediated knockdown, HeLa cells were kept under basal conditions (panela, scale bar, 25 μm) or treated with 200 μm CuCl2for 5 h (panelb, scale bar, 25 μm), and then fixed, immmunostained with antibodies against ATP7A (green) and TGN46 (red) and analysed by confocal microscopy. (c) Percentage of cells with ATP7A in the TGN following the copper treatment (left panel). Intensity of ATP7A signal in the TGN was quantified using Image J (right panel). (d) ANKRD9 knockdown results in fragmented TGN and fragmented ATP7A staining pattern. Following siRNA-mediated knockdown, HeLa cells in basal conditions were fixed, stained with antibodies against ATP7A (green) and TGN46 (red) and analysed by confocal microscopy. Scale bar, 25 μm. Analysis of the knockdown genes that produced copper elevation with the z -scores above 3 revealed a role for lipid metabolism in maintenance of copper levels ( Supplementary Table 5 ). This observation is especially interesting, because our previous studies in the animal model of copper overload demonstrated that accumulating copper specifically downregulates lipid metabolism. Finally, our screen suggested which transporters might be used for the uptake and removal of zinc from HeLa cells [28] , [29] . For example, within the ZnT and Zip family members, knockdown of ZIP1 ( z -score of 6.07) mostly increased zinc level, whereas knockdown of ZIP5 ( z -score of 3.09) decreased it. Overall, our data demonstrated that the siRNA screen can identify regulators of trace elements in human cells and predict key regulatory mechanisms. Pathway analysis of selenium distribution We subjected the candidates from the screen to several gene network analysis tools: DAVID pathway analysis [30] , protein–protein interactions using STRING database [31] , GeneSifter (Geospiza) and IPA INGENUITY pathway analyses. In the case of selenium, using DAVID, we observed a significant functional cluster of ribosomal proteins (the Fisher exact test, P =8.94 × 10 −3 ; Benjamini P value adjustment, P =0.36; all results were derived from three replicates). Table 2 lists genes associated with this cluster. This observation is consistent with the finding that the knockdowns of several ribosomal genes led to an increase in selenium levels in HeLa cells ( Fig. 3a ). Notably, the shape of ionomic profiles was similar for all these knockdown conditions ( Fig. 3a ) and it was different from that of other targets (for example, glycolytic enzymes: GAPDH, PGK1 and PGM1). We further performed structural analysis of this functional cluster and observed that most of the identified ribosomal proteins (11 of 14) were located at the interface of two ribosomal subunits near the transfer RNA-binding site ( Fig. 3b ). It is possible that deficiency in these ribosomal proteins alters the ribosome structure facilitating an increased Sec insertion. It is also possible that these knockdowns decreased the rate of protein synthesis, which indirectly supported the inherently slow Sec insertion. Our data point to a global control of selenoprotein expression through ribosome structure and function. The specific mechanism of this control requires further studies. Table 2 Cluster of ribosomal genes identified as selenium regulators. Full size table Figure 3: Characterization of genes that affect the selenium ionome. ( a ) Ionomic profile data of the ribosomal functional cluster. Selenium z -scores (derived from three replicates) from the screen were analysed by using DAVID. Glycolytic enzymes (GAPDH, PGK1 and PGM1) are shown for comparison. ( b ) Model of eukaryotic (yeast) 80S ribosome with the location of identified ribosomal cluster genes. ( c ) Analysis of selenium candidates in HeLa cells by metabolic 75 Se labelling. HeLa cells were transfected with the indicated siRNAs. 75 Se was added to the cells 24 h before harvesting. Cell lysates were analysed by SDS–polyacrylamide gel electrophoresis followed by western blotting with antibodies specific for selenoprotein S and β-actin. The 75 Se-labelling pattern was visualized with a PhosphorImager. Full size image We further analysed selected selenium candidates with high z -scores: nuclear RNA export factor (its knockdown increased selenium in cells), ribosomal protein L14 (RPL14; its knockdown increased selenium) and potassium voltage-gated channel, member A1 (KCNA1; its knockdown decreased selenium). We also included SBP2 as a Sec machinery component identified in the screen. HeLa cells transfected with these siRNAs were metabolically labelled with 75 Se ( Fig. 3c ) and gene knockdowns verified by real-time PCR ( Supplementary Fig. 3 ). RPL14 and KCNA1 siRNAs differentially affected selenoprotein expression: RPL14 deficiency increased the levels of selenoproteins TR1 (a major 55 kDa band detected by 75 Se labelling) and selenoprotein S (detected by western blotting), whereas KCNA1 deficiency decreased the expression of several selenoproteins with the molecular weight under 25 kDa. The SBP2 siRNA decreased the expression of all selenoproteins. Overall, the data pointed to several genes whose knockdown affected selenium levels in HeLa cells owing to changes in selenoprotein expression. Two of these genes ( RPL14 and KCNA1 ) have not been previously linked to selenium metabolism. Target validation revealed new regulators of ATP7A Our validation analyses revealed several candidates not known previously to be involved in the regulation of trace element homoeostasis ( Table 1 ). Knockdowns of two members of the DNAJ family (DNAJC5 and DNAJC17), two kinase inhibitor genes ( CAMK2N2 and IBTK ) and two transporters (SLC6A4 and ABCC3) led to increased copper levels ( Table 1 ). To uncover specific roles of these genes in a cellular copper balance, we determined the effects of their inactivation on ATP7A, the major copper export protein in HeLa cells. Following downregulation of the target genes, we characterized ATP7A expression, intracellular targeting and its ability to undergo copper-dependent trafficking from trans -Golgi network (TGN) to the plasma membrane (a step required for copper efflux). Out of seven tested targets, downregulation of five had a significant effect on ATP7A. This result emphasizes the primary role of ATPase-mediated copper export in balancing cellular copper. Knockdown of DNAJC5 and SLC6A4 did not influence ATP7A protein levels, trafficking or targeting, indicating that these proteins may regulate other components of the copper-handling machinery. In contrast, knockdown of a member of the HSP40 family DNAJC17 produced a significant reduction in ATP7A amount in cells as evidenced by the decreased intensity of ATP7A signal (green) in the TGN compared with the marker TGN46 (red; Fig. 4a , Supplementary Fig. 4 ). The decrease of ATP7A in the TGN was due to lower ATP7A protein levels (rather than the loss of TGN targeting) as evidenced by western blotting of cellular lysates ( Fig. 4b ). The levels of other tested proteins, such as Na,K-ATPase and TGN46, were not affected. By comparing the effects of the siRNA pool and four individual anti-DNAJC17 siRNAs, we determined that the effect of DNAJC17 inactivation on ATP7A levels might be indirect, since the same degree of DNAJC17 downregulation by different siRNA yielded different changes in the ATP7A levels (see Methods for details). Knockdowns of the kinase inhibitors IBTK (inhibitor of Bruton tyrosine kinase) and CAMK2N2 (calcium/calmodulin-dependent protein kinase II inhibitor 2) had a dual effect: reduction in the ATP7A levels and a downwards shift in the ATP7A electrophoretic mobility ( Fig. 4 ; Supplementary Fig. 4 ) that suggested changes in the post-translational modification of ATP7A. Figure 4: Characterization of targets that affect copper levels in HeLa cells. ( a ) Effect of targets downregulation on ATP7A localization in basal conditions. Following gene-specific siRNA-mediated knockdowns, HeLa cells were fixed, stained with the antibodies against ATP7A (green) and the TGN marker TGN46 (red) and analysed by confocal microscopy. The merged image is shown in the right panel. Scale bar, 25 μm. ( b ) Effect of target downregulation on ATP7A protein levels and electrophoretic mobility. Following gene knockdowns, HeLa cell lysates were analysed by western blotting. The blot was cut at 130 kDa; the upper part was immunostained for ATP7A and the lower part was immunostained for Na/K-ATPase. A representative blot is shown; the entire blot is included as Supplementary Fig. 6 . ( c ) Quantification of western blot data by densitometry. The ATP7A protein levels were normalized to Na/K-ATPase protein levels and the values were compared with the intensity of ATP7A in cells transfected with a non-targeting siRNA (scrRNA). The error bars correspond to s.d. values from four independent experiments. Asterisks mark significant changes (the Mann–Whitney U -test, P <0.05; lower panel). Full size image A different mode of ATP7A regulation was detected in the case of the ABCC3 knockdown. Downregulation of this gene did not have a significant effect on ATP7A levels ( Fig. 4b ) or ATP7A targeting to the TGN ( Fig. 5a ). Instead, in cells with the downregulated ABCC3 (ATP-binding cassette, subfamily C (CFTR/MRP), member 3) the distribution of ATP7A between the TGN and vesicles was altered, with less ATP7A leaving the TGN in response to copper treatment ( Fig. 5b,c ). Perhaps, the most intriguing results were obtained with cells depleted of ANKRD9. Downregulation of this adaptor protein led to an increased cell size, dispersion of the TGN ( Fig. 5d ) and a change in ATP7A electrophoretic mobility ( Fig. 4b ). A shift in ATP7A migration on SDS–polyacrylamide gel electrophoresis ( Fig. 4b ) suggests that the post-translational modifications of ATP7A, which is a glycosylated protein, are affected. Although the ANKRD9 knockdown affected TGN morphology, it did not disrupt co-localization of ATP7A and TGN46, suggesting that the molecular identity of this compartment was preserved ( Supplementary Fig. 4b ). We are now facing intriguing mechanistic questions about a link between TGN morphology, ATP7A modification and cellular copper levels. Taken together, these data show that essentially all effects of the target gene knockdowns with respect to copper elevation can be explained by changes in ATP7A trafficking, modification and/or expression. Cellular machinery that controls ATP7A mRNA and/or protein stability has not been previously characterized, and the identification of several new regulatory components as a result of the ionomics screen provides exciting opportunities for better understanding of copper metabolism in human cells. Figure 5: ABCC3 and ANKRD9 are new regulators of ATP7A. ( a – c ) Downregulation of ABCC3 affects ATP7A trafficking. Following siRNA-mediated knockdown, HeLa cells were kept under basal conditions (panel a , scale bar, 25 μm) or treated with 200 μm CuCl 2 for 5 h (panel b , scale bar, 25 μm), and then fixed, immmunostained with antibodies against ATP7A (green) and TGN46 (red) and analysed by confocal microscopy. ( c ) Percentage of cells with ATP7A in the TGN following the copper treatment (left panel). Intensity of ATP7A signal in the TGN was quantified using Image J (right panel). ( d ) ANKRD9 knockdown results in fragmented TGN and fragmented ATP7A staining pattern. Following siRNA-mediated knockdown, HeLa cells in basal conditions were fixed, stained with antibodies against ATP7A (green) and TGN46 (red) and analysed by confocal microscopy. Scale bar, 25 μm. Full size image A previous study by Yu et al. [21] yielded a detailed summary of ionomic changes in a full-genome collection of Saccharomyces cerevisiae single-gene deletion strains. Since key metal-handling molecules are conserved in yeast and human cells, we compared the effects of yeast knockouts and HeLa knockdowns of experimentally confirmed and new regulators identified in the screens. Unexpectedly, the comparison of mammalian and yeast metalloregulons showed little overlap in the identity of proteins affecting metal balances. Specifically, the consequence of 25 yeast knockouts (18 genes identified as influencing copper levels and 7 altering iron levels) were similar only for three orthologues in HeLa cells: NPP2/ENPP6 and GRR1/FBXL15 pairs of orthologues showed similar effects on copper levels and the MET30/FBXW2 pair was similar with regard to iron ( Supplementary Table 6 ). Given this observation, we compared the effects of deletions of genes with firmly established roles in copper homoeostasis, that is, yeast yCTR1, ATX1, yCCS and CCC2 with those of human hCTR1, ATOX1, hCCS and ATP7A. Downregulation of the high-affinity copper uptake transporter yCTR1/hCTR1 was associated with a decrease in cellular copper content in both yeast and mammalian cells. However, consequences of the deficiency in the three other genes differed, not only in value but also in the direction of change ( Table 3 ). Inactivation of ATP7A, CCS and ATOX1 in HeLa cells (our screen) produced effects that were consistent with the established physiological functions of these proteins. Dissimilar results in yeast may reflect the cell adaptation to stable gene deletion (in contrast to the siRNA-mediated knockdown that produced transient gene inactivation in HeLa cells) or different growth/medium conditions. It is also possible that copper metabolism in yeast is regulated primarily by copper uptake, while in HeLa cells copper balance is largely controlled by copper export. Table 3 Effects of inactivation of orthologous genes corresponding to major copper regulators in yeast and HeLa cells. Full size table In this study, we identified new regulators of trace elements in human cells and uncovered fundamental differences in how levels of trace elements are controlled. This was achieved through a high-throughput siRNA/ICP-MS screen in which the levels of trace elements were determined following knockdown of 21,360 genes in HeLa cells. Automation of ICP-MS analysis and the custom use of a high-throughput sample delivery system allowed rapid, reliable and cost-effective profiling of trace elements. In our system, 1,080 samples could be processed every 24 h using a single instrument and more than 30,000 samples per month. The entire human genome siRNA library was analysed in triplicate in just 100 days. The result is the first high-throughput ionomics study in mammalian cells. Earlier ionomics analyses were mostly carried out using a S. cerevisiae knockout collection [17] , [18] . S. cerevisiae shares key components of the machinery regulating copper, zinc and iron metabolism with mammals; however, our data indicate that the contribution of these and other regulators to overall metal ion balance may differ between yeast and mammalian cells. Moreover, S. cerevisiae does not utilize several trace elements used by mammals. These results highlight the importance of verifying findings in model systems in human cells, especially for fine aspects of regulation. We did not supplement the growth medium with trace elements, since the necessary metal ions were already present in the calf serum at sufficient levels, and our aim was to identify proteins that modulate trace elements under normal growth conditions. Our approach, however, can be extended to other conditions (such as cells subjected to trace element supplementation or metabolic perturbations) and more complex cell systems (such as specialized cells or polarized cell layers). The screen was carried out in triplicate and utilized the same batches of cells, media, buffers and the digestion mix. The results provide many valuable avenues for further studies. We found that most gene knockdowns in HeLa cells changed levels of one and rarely more than one element. By comparison, the ionomics study of yeast gene deletions detected 210 strains with significant changes in at least one element [18] , and the majority of these strains showed changes in several elements. Detailed interpretation of the findings is not straightforward in either yeast or human cells and will require additional studies and screens. It was suggested that linear mixed-effect models could help reduce noise in genome-wide perturbation screens including ionome studies [32] . In the future, advanced statistical models may help identify and refine predictions of new candidate genes regulating elemental composition of cells. Our results suggest that the trace elements are regulated largely independently. We also observed fundamental differences in the modes of regulation of different trace elements in human cells. Thus, the selenium ionome is controlled by retaining this element in the cell via insertion into selenoproteins. Dysregulation of this process appears to lead to selenium excretion, since deficiency in either a limiting factor in Sec insertion or the most abundant selenoprotein decreased selenium in cells. On the other hand, dysfunction in ribosome function increased cellular selenium. This observation suggests that selenoprotein levels rather than selenium levels may serve as a signal for regulation. The state of the copper ionome strongly depends on the presence of copper exporter (ATP7A in HeLa cells) and the machinery that controls its maturation and function. Consequently, the most common phenotype of knockdown conditions was copper elevation. The iron ionome showed a third pattern, with many knockdown conditions slightly changing the levels of this element, and the only large effect was observed under conditions that interfered with iron transferrin receptor-mediated import. We also observed significant differences in the stability of various ionomes. Among trace elements, the zinc ionome was the most stable, whereas copper levels could be more easily changed in cells. In the follow-up study, we characterized the genes predicted to be involved in selenium and copper metabolism (this focus was because of the expertise of the contributing laboratories; we hope that additional targets will be examined in future studies by our or other groups). With regard to selenium, the selenoprotein TR1 (Rundlof and Arner [33] ) was one of the top selenium hits in the screen. This was unexpected as the human genome has 25 selenoprotein genes, and the most abundant mammalian selenoprotein is GPx1. By taking advantage of the fact that all mammalian selenoproteins that function inside cells have a single Sec, we used metabolic 75 Se labelling to show that TR1 is the most abundant selenoprotein in HeLa cells. Thus, the ICP-MS approach was highly sensitive: deficiency in just one selenoprotein significantly decreased the levels of cellular selenium. Another selenium target was SBP2. Subsequent analyses revealed that SBP2 deficiency led to a decrease in the expression of all selenoproteins in HeLa cells. Other components of the Sec machinery were not detected, suggesting that SBP2 is the limiting factor in Sec incorporation in HeLa cells. We also identified new genes that regulate selenium metabolism. Knockdown of potassium voltage-gated channel (KCNA1) decreased selenium levels, which may represent a direct or indirect effect. In addition, knockdown of a ribosomal structural protein RPL14 resulted in an increased selenium level and an increased expression of TR1 and selenoprotein S. Moreover, several ribosomal proteins showed a very similar ionomic phenotype, with selenium being the most affected among all tested elements. Most of these proteins localized to the interface between the two ribosomal subunits. The Sec incorporation system includes several protein factors, a Sec transfer RNA, and a specific mRNA structure, the SECIS element [34] . Reduced expression of ribosomal proteins may lead to structural changes in the ribosome that affect Sec insertion. It is also possible that this condition decreases the rate of protein synthesis, which may indirectly increase the inherently slow Sec insertion. Several genes known to be involved in homoeostasis of trace elements, such as ATP7A, ATOX1 and MT1A (copper), and TFRC (iron), ZIP1 and ZNT5 (zinc), produced changes in the levels of respective elements. The knockdown of the copper exporter ATP7A led to the most significant increase in copper levels as expected from previous reports [9] , [35] . The knockdown of another copper-exporting ATPase, ATP7B, did not change copper levels, most probably because of the low ATP7B expression in HeLa cells [36] . Downregulation of SLC31A1 (hCTR1), the high-affinity copper importer in mammalian cells [9] , only slightly decreased copper levels, presumably because of the availability of certain low affinity uptake systems [37] . The identity of the low affinity copper transporter is unknown; however, our screen identified several candidate transporters, including Zip5, which lowered copper levels when downregulated. In addition, metallothionein (MT1A) was as an important player in balancing copper under basal conditions. This result is unexpected as metallothioneins are thought to be involved in sequestration of excess copper [38] . In addition to the already known proteins, our screen revealed new regulators of copper homoeostasis. Knockdowns of IBTK, CAMK2N2, DNAJC5, DNAJC17, ABCC3, ANKRD9 and SLC6A4 resulted in elevation of intracellular copper. Both IBTK and CAMK2N2 are kinase inhibitors, and their downregulation resulted in a significant decrease in ATP7A protein levels. Kinase-mediated phosphorylation plays a role in the trafficking of ATP7A (Voskoboinik et al. [39] and Veldhuis et al. [40] ; however, roles of Bruton tyrosine kinase or CAMK2 in ATP7A phosphorylation have not been previously known or considered. It is interesting that both kinases participate in major signalling pathways involving a nuclear factor-kappaB [41] , [42] , [43] . These results suggest a link between the stress–response pathways and a tight regulation of copper homoeostasis. The negative effect of ABCC3 downregulation on ATP7A trafficking is an equally novel result. ABCC3 is an organic anion and bile-acid transporter. Previously, treating hepatocytes (HepG2) with copper resulted in an upregulation of ABCC3 (Song et al. [44] ). Together, these results suggest that the bile-acid transport and copper metabolism might be linked. The observed increase in copper levels in response to dysregulation of lipid metabolism further supports the idea of copper and lipid homoeostasis being functionally interconnected. The downregulation of ABCC3 may also be affecting the organic anion/bile-acid balance in HeLa cells, which might inhibit ATP7A transport activity and copper-responsive trafficking, which are also mutually dependent. Downregulation of ANKRD9 (ankyrin repeat domain-containing protein 9) produces a complex phenotype, which includes fragmented TGN and apparent changes in ATP7A post-translational modification and protein levels. The function of this protein is not known, but it was suggested to play a role in lipid metabolism [45] . Other ankyrin proteins are involved in membrane protein trafficking/stabilization [46] , [47] . Thus, ANKRD9 may bind to ATP7A and stabilize its TGN localization. Furthermore, ANKRD9 induced a decrease in ATP7A protein levels and a shift in ATP7A migration on SDS–polyacrylamide gel electrophoresis, which could be a secondary effect of TGN fragmentation and may alter the ability of ATP7A to efficiently pump excess copper out of the cell. In conclusion, we developed a sensitive high-throughput method to profile trace elements in mammalian cells on a genome-wide scale using ICP-MS. A total of 21,360 human gene knockdowns were analysed for changes in trace elements in HeLa cells. This approach detected many known genes involved in transport and regulation of trace elements, and identified novel genes that regulate the metabolism of selenium and copper. More generally, this study uncovered fundamental differences in the regulation of trace elements. Our results offer a valuable data set that could be further used experimentally and mined by the broader research community to uncover novel trace element-dependent genes and processes. Cell culture and screening conditions Comparative analysis of several human cell lines (HEK 293, HTC 116, Caco2 and HeLa, obtained from American Type Culture Collection) was carried out with regard to their attachment and resistance to washing. HeLa cells were chosen for subsequent experiments, because they had higher levels of most analysed trace elements, showed high transfection efficiency and sustained extensive washing ( Supplementary Fig. 5A ). The human siGenome library from Thermo Fisher Scientific (formerly Dharmacon) was used in the study. The siRNA screening procedure was based on the Dharmacon’s Wet Reverse Transfection Protocol, version 2.0. Modifications were made for use with HeLa cells. siRNA pools targeting 21,360 genes were used with 267 96-well plates. Eighty such pools, transfected at 20 nM per well final concentration, were used per plate. On the day of transfection, plates (96-well, V-bottom) with siRNA pools were removed from the −80 °C freezer and allowed to warm to room temperature. OptiMEM medium and Dharmafect 1 reagent (final concentration 0.13 μl per well) were added using Thermo Multidrop Micro liquid dispenser. Plates were placed on an orbital shaker for 20 min at room temperature. Using a Biomek FX mixer (Beckman Coulter), each master plate was mixed two times and 20 μl of the siRNA/DF1/OptiMEM complex was transferred to each well of the tissue culture plate. After completion of the transfer, HeLa cells were dispensed (2.5 × 10 4 cells per well). Total transfection volume was 100 μl. Immediately after plating, each set of plates was placed at 37 °C in a 5% CO 2 incubator. ICP-MS analysis Approximately 72 h after transfection, HeLa cells were washed and acid digested. Medium was removed using a Biomek FX liquid-handling station. Plates were rapidly washed three times with 100 μl per well of TE buffer (10 mM Tris pH 7.4, 1 mM EDTA). We tested several washing buffers previously used in ICP-MS studies (HEPES-bicarbonate, HEPES-citrate and TRIS-EDTA (TE), all at pH 7.4) [48] , [49] for optimal removal of the contaminating elements before acid digestion and ICP-MS analysis ( Supplementary Fig. 5B ). Cells rapidly washed with TE buffer repeatedly showed the most stable and consistent elemental signals, so this buffer was chosen for the siRNA screen. Digestion mix (100 μl per well) was added to all wells and contained 1.5% nitric acid (w/v), 1.5% hydrogen peroxide (w/v) and 50 p.p.b. Ga as an internal standard. Finally, plates were placed in a humidified incubator at 70 °C for 2 h. All digested plates were sealed to prevent evaporation and stored at −80 °C until ICP-MS analysis. ICP-MS analyses were performed at the University of Nebraska-Lincoln Spectroscopy core facility equipped with Agilent Technologies ICP-MS 7500cs (Santa Clara, CA) and a ESI SC-4 high-throughput autosampler (Elemental Scientific Inc., Omaha, NE). The unit could accommodate six 96-well plates. The SC-Fast sample introduction system was modified to allow analysis of 100 μl samples by using a microperipump (MP-2) to push the carrier solution (1.5% nitric acid) through an injection loop (70 μl) at a flow rate of 70 ml min −1 . A second microperipump (MP-1) was used to rinse the sample loop and load the samples onto the injection loop within 8–10 s. The analysis used the octopole collision cell filled with 3.5 ml min −1 of hydrogen gas and 1.5 ml min- of helium with an argon carrier flow of 0.9 l min −1 and argon make-up flow of 0.15 l min −1 , and RF power of 1,500 W. An ICP-MS method was optimized for the analysis of 18 elements ( 7 Li, 11 B, 23 Na, 24 Mg, 31 P, 34 S, 39 K, 40 Ca, 55 Mn, 56 Fe, 59 Co, 60 Ni, 63 Cu, 66 Zn, 75 As, 78 Se, 95 Mo and 111 Cd) in HeLa cells, with 71 Ga as the internal standard. Calibrations were performed after analysing ~3,000 samples. Instrument performance was verified by spiking a blank with 10% of the standard stock mix. Replicate samples were on different plates, in which individual knockdowns were located in the same position (well on the plate). Data normalization and analysis The data processing procedure is summarized in Supplementary Fig. 2 . First, we manually checked the ICP-MS signal for each element in each plate (nine experimental elements and phosphorus). For each element, to subtract noise, the average value of the five background wells (individual outliers were identified and removed using Dixon’s Q-test) was subtracted from the original signal for each gene knockdown in each plate replicate. Second, in each plate, we used the average value of the control samples (scrambled non-targeting RNA, scrRNA, outliers were also removed) to normalize signals for all genes. As there were three replicates for each gene, normalized signals in each replicate were sorted and outlier values were further removed (Dixon’s Q-test). Third, an algorithm was developed that removed additional biases, including those associated with ‘row slope’ effect (the signals of genes in one column were significantly different from other columns for multiple elements) and cell number. The first bias was corrected based on the average value of each column of a plate. The second bias was corrected using the average of phosphorus, manganese, selenium and zinc signals that appeared to be the most stable signals among all elements analysed. For the resulting normalized data set, we used the average values of each gene from the replicates and calculated fold change and the z -score that measures distances between the signal for each gene and the average signal for all genes within the same plate (number of s.d. from the mean). The prediction intervals for elements were as follows: Mg (−3.33,3.34), P (−3.36,3.36), K (−3.32,3.32), Mn (−3.34,3.34), Fe (−3.33,3.32), Cu (−3.34,3.34), Zn (−3.35,3.35), Se (−3.34,3.35) and Cd (−3.30,3.30). The data are available through the following website: http://www.gladyshevlab.bwh.harvard.edu/ICPMS_Human . RNA isolation and quantitative PCR To evaluate the efficiency of siRNA knockdown in HeLa cells, we performed real-time PCR analyses. HeLa cells were transfected with the indicated siRNA or scrRNA control. Complementary DNA was obtained using a Cells-to-cDNA kit (Ambion). Genomic DNA was removed using a DNA removal kit (Ambion). Complementary DNA was obtained using the oligo dT primer. Real-time PCR was performed using a Fast SYBR Green master mix (Applied Biosystems). Primer sequences for the expression analysis were as follows: KCNA1, 5′-TTCTTCGACCGCAACCGGCC-3′ and 5′-AGCTATCTCGGTGCCCAGGGT-3′; RPL14, 5′-AGGTTGGCCGGGTGGCCTAT-3′ and 5′-AGGCGCTGCTTTCTGGCCTG-3′; SBP2, 5′-GCAGGCAGAGCTGTCAGGGC-3′ and 5′-TGGGCTCTCCCACCAGCTCC-3′. Special 18S ribosomal RNA-modified primers (Ambion) were used as an internal control for data normalization. We also compared the consequence of downregulation with the individual and pooled DNAJC17 siRNAs, since knockdown of this gene showed the strongest effect on ATP7A levels. These studies revealed that only one individual siRNA (#2) decreased the ATP7A levels similar to the pool, whereas other individual siRNA (and a combination of three out of four, #1, #3 and #4) had no significant effect on ATP7A levels despite a significant decrease in the mRNA levels for DNAJC17 (confirmed by real-time PCR). Thus, the effect of DNAJC17 knockdown on ATP7A may be indirect or confounded by other unknown factors. X-ray fluorescence microscopy HeLa cells were grown on 2 × 2 mm 2 silicon nitride windows (Silson, Blisworth, UK) and transfected with siATP7A or scrRNA control. Seventy-two hours after transfection, cells were washed three times in PBS (pH 7.4) and fixed in 4% formaldehyde in PBS for 15 min. Windows were air dried for elemental imaging. Samples were stored at room temperature until analysis. Trace elements were mapped at the beamline 2-ID-E, advanced photon source, Argonne National Laboratory (Argonne, IL) using a hard X-ray microprobe (6–30 keV). Images were obtained by raster-scanning with resolution of 1 μm. Full X-ray fluorescence spectra were recorded for each pixel using energy-dispersive Vortex detector (SII Nanotechnologies, Northridge, CA). For quantification, thin film standards NBS-1832 and NBS-1833 (National Bureau of Standards, MD) were used. Western blotting and immunohistochemistry Modified version of the Dharmacon’s Wet Reverse Transfection Protocol was used for the transfection of HeLa cells. Dharmafect I reagent (0.4 μl per well) was diluted using OptiMEM media (24.6 μl per well). Stock siRNA was mixed with OptiMEM to a final volume of 10 μl (the final siRNA concentration is 20 nM per well). Both Dharmafect I/OptiMEM and siRNA/OptiMEM solutions were mixed and added to each well of an 8-well chamber (Millipore). Chambers were incubated for 30 min at room temperature. HeLa cells were trypsinized and resuspended in antibiotic-free complete medium. Cells (0.3 × 10 5 ) were added to each well in a volume of 170 μl. The chambers were placed at 37 °C in a 5% CO 2 incubator. Sixty hours after the transfection, 200 μl of antibiotic-free complete medium was added to each well. Cells were fixed 72 h after the transfection using 3% paraformaldehyde at 37 °C for 12 min. Cells were washed with 1 × PBS and blocked/permeabilized simultaneously for 12 min using 0.1% BSA/0.1% saponin in 1 × PBS. Cells were washed with 1 × PBS and then incubated with appropriate primary and secondary antibodies diluted in 0.1% BSA in 1 × PBS (primary antibody: mouse anti-ATP7A antibody 1:250 (Santa Cruz) and sheep anti-TGN46 1:300 (Genetex). Secondary antibody: Alexa Fluor 488 goat anti-mouse antibody 1:500 (Invitrogen) and Alexa Fluor 555 donkey anti-sheep 1:500 (Invitrogen). The glass slides were mounted using Fluoromount G w/DAPI (Electron Microscopy Sciences). Images were taken using a Zeiss LSM 510 confocal microscope and a 40X oil immersion objective. For western blotting, cells were harvested, the pellet was resuspended in 30 μl of Laemmli loading buffer, sonicated for 30 s and centrifuged for 15 min at 3,000 g at 4 °C. The supernatant was loaded to 8% SDS gel. Proteins were transferred to a polyvinylidene difluoride membrane using CAPS buffer, pH 11.0. The membrane was cut at 130 kDa and probed for Na/K-ATPase (1:10,000; Millipore) and ATP7A (1:3,000; Santa Cruz). Goat anti-mouse IgG-HRP (1:10000, Santa Cruz) was used as a secondary antibody and the membranes were developed using a SuperSignal West Pico Substrate (Thermo Scientific). How to cite this article: Malinouski, M. et al. Genome-Wide RNAi ionomics screen reveals new genes and regulation of human trace element metabolism. Nat. Commun. 5:3301 doi: 10.1038/ncomms4301 (2014).